Genomic mapping of phosphorothioates reveals partial modification of short consensus sequences Bacterial phosphorothioate (PT) DNA modifications are incorporated by Dnd proteins A-E and often function with DndF-H as a restriction-modification (R-M) system, as in Escherichia coli B7A. However, bacteria such as Vibrio cyclitrophicus FF75 lack dndF-H , which points to other PT functions. Here we report two novel, orthogonal technologies to map PTs across the genomes of B7A and FF75 with >90% agreement: single molecule, real-time sequencing and deep sequencing of iodine-induced cleavage at PT (ICDS). In B7A, we detect PT on both strands of G ps AAC/G ps TTC motifs, but with only 12% of 40,701 possible sites modified. In contrast, PT in FF75 occurs as a single-strand modification at C ps CA, again with only 14% of 160,541 sites modified. Single-molecule analysis indicates that modification could be partial at any particular genomic site even with active restriction by DndF-H, with direct interaction of modification proteins with GAAC/GTTC sites demonstrated with oligonucleotides. These results point to highly unusual target selection by PT-modification proteins and rule out known R-M mechanisms. Secondary modifications of DNA and RNA play critical roles in cell physiology, including restriction-modification (R-M) systems in prokaryotes, and in epigenetic control of DNA replication, transcription and translation in all organisms [1] . While the incorporation of sulphur (S) into nucleobases is well established in secondary modifications of transfer RNA (tRNA) and ribosomal RNA (rRNA) [2] , the replacement of a non-bridging phosphate oxygen with sulphur as a phosphorothioate (PT) was originally developed as an artificial means to stabilize oligodeoxynucleotides against nuclease degradation [3] . We recently discovered that the dnd gene products incorporate sulphur into the DNA backbone as a PT in a sequence- and stereo-specific manner [4] , [5] . Beginning with the original observation in Streptomyces lividans that the five-gene dnd cluster ( dndA-E ) caused DNA degradation during electrophoresis [6] , [7] , [8] , the presence of dnd genes and PT modifications has been established in >200 different bacteria and archaea, including many human pathogens [6] , [9] , [10] , [11] , [12] , [13] , [14] , [15] . However, the functional landscape of PT modifications has not been firmly established. At the biochemical level, an emerging picture of Dnd protein function reveals that DndA acts as a cysteine desulfurase similar to Escherichia coli lscS and assembles DndC as a 4Fe-4 S cluster protein [16] . More than half of dnd gene clusters lack dndA and contain only dndB-E , with DndA cysteine desulfurase activity functionally replaced by a host gene linked to the dndB-E cluster (for example, E. coli IscS) [17] . DndC possesses ATP pyrophosphatase activity and is predicted to have PAPS reductase activity, while DndB is predicted to have a domain for binding Fe-S cluster proteins, as well as homology with a DNA repair ATPase and with transcription regulators [6] , [9] . A DndD homologue in Pseudomonas fluorescens , SpfD, has ATPase activity possibly related to DNA structure alteration or nicking during PT incorporation [18] . Finally, the DndE structure reveals a tetramer conformer and a possible nicked double-strand DNA binding protein [19] . In terms of higher function of the dnd genes and PT modifications, there is evidence that in some bacteria, PT modifications are part of a novel R-M system with similarities to methylation-based R-M systems [20] , [21] , such as sequence specificity and discrete levels associated with 4-6 nucleotide consensus sequences [4] , [5] . We recently identified a restriction system comprised of a 3-gene family, dndFGH , the products of which cleave DNA lacking sequence-specific PT modifications [22] , [23] . By BLAST searching, ~86 bacterial strains have been found with both dndA-E and dndF-H co-localized on the same mobile genetic element. However, there are ~125 bacterial strains lacking the dndF-H restriction system in spite of possessing dndA-E and PT. The fact that many strains of bacteria lack the restriction enzyme component of a typical R-M system is consistent with the idea that PT modifications and dndA-E genes provide functions other than R-M, such as control of gene expression. To better understand PT biology, we place the modifications in the context of the genomic landscape by developing two highly novel, orthogonal technologies to quantitatively map PT locations in bacterial genomes: single-molecule, real-time (SMRT) sequencing [24] , [25] , [26] , [27] , [28] and deep sequencing of iodine-induced cleavage at PT (ICDS) ( Fig. 1 ). These methods are then applied to two bacterial strains known to possess PT modifications with different features. With regard to PT function in an R-M system, E. coli B7A possesses both the modification genes ( dndB-E ) and the restriction genes ( dndF-H ), with PT modifications occurring in G ps A and G ps T contexts at 370±11 and 398±17 PT per 10 6 nucleotides, respectively [5] . This is consistent with an R-M consensus sequence of G ps AAC/G ps TTC, as observed in the related Salmonella enterica [22] . However, the frequency of PT modifications in this genome (~1 per 2,500 nt) is too low to account for a four-nucleotide consensus sequence expected to occur once in every ~300 nt by chance alone. In terms of PT functions other than R-M, many bacteria, such as Vibrio cyclitrophicus FF75, lack the restriction genes dndF-H , which points to other roles such as epigenetic control of gene expression. PT modifications in FF75 occur in C ps C contexts at a frequency of 2,600±22 per 10 6 nt, or once in every 380 nt [5] . We provide a genomic context for these fragmentary observations by developing and applying the SMRT and ICDS technologies to obtain the first high-resolution genomic maps of PT modifications, with the discovery of highly unusual and unexpected features of this DNA modification. 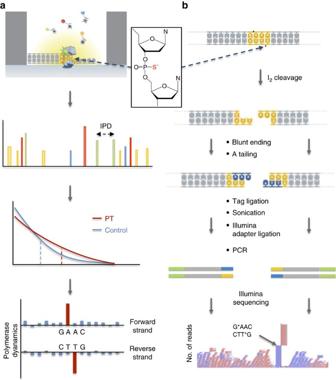Figure 1: Schematic illustrations of the two approaches to sequence mapping of PT modifications. An example of a PT-modification structure is shown in the inset. (a) SMRT sequencing and (b) ICDS methods. Figure 1: Schematic illustrations of the two approaches to sequence mapping of PT modifications. An example of a PT-modification structure is shown in the inset. ( a ) SMRT sequencing and ( b ) ICDS methods. Full size image Genome sequencing of E. coli B7A and V. cyclitrophicus FF75 The first step in mapping PT modifications was to define the complete genome sequences for B7A and FF75. The V. cyclitrophicus FF75 genome was originally sequenced using the Illumina platform, yielding 77 contigs (GenBank number AIDE00000000) [29] . To complete the sequencing, we made a large randomly fragmented SMRTbell library with an average insert size of ~10 kb and sequenced the library by SMRT using the XL long-read length polymerase. The assembly was completed using a recently developed algorithm, HGAP [30] , which yielded five large contigs for a total of 5.1 Mb. Based on the assembly and sequenicng coverage analysis, there appear to be two circular chromosomes, which is similar to other Vibrio species [31] . One of the two Vibrio chromosomes assembled to completion, the other was broken into four contigs by several large repeats that were too large to be spanned by long reads. The contigs were annotated by RAST, submitted to NCBI and assigned to Genbank ID ATLT00000000. The B7A genome was similarly sequenced using the SMRT platform and the annotated genome is presented in Supplementary Data 1 . An ~10 kb fragment library, 8 SMRT cells and HGAP de novo assembly were used to complete the whole-genome sequence as a single, circular chromosome of 4,944,397 bases, 5,031 orfs, 22 rRNAs and 86 tRNAs. There were also four circular plasmids: pEB1 - 89,507 bases, 107 orfs; pEB2 - 52,028 bases, 67 orfs; pEB3 - 66,341 bases, 85 orfs; pEB4 - 78,167 bases, 94 orfs. The GenBank accession numbers for the chromosome and plasmids are CP005998 , CP005999 , CP006000 , CP006001 and CP006002 , respectively. Adaptation of SMRT sequencing to map PT modifications The SMRT DNA sequencing platform uniquely detects DNA modifications by virtue of variations in the interpulse duration (IPD) of the DNA polymerase kinetics [26] , with initial applications related to nucleobase methylation [26] , 5-hydroxymethylcytosine [28] and damaged nucleobases [25] . To test the feasibility of SMRT sequencing for the detection of PT modifications in DNA, we designed synthetic 20-mer oligodeoxynucleotides containing sequence-specific PT in the R p or S p configuration and compared the IPD with unmodified templates. As shown in Fig. 2a , the presence of a PT resulted in a readily detectable kinetic signal at the modification site, but interestingly only for the naturally occurring R p configuration. 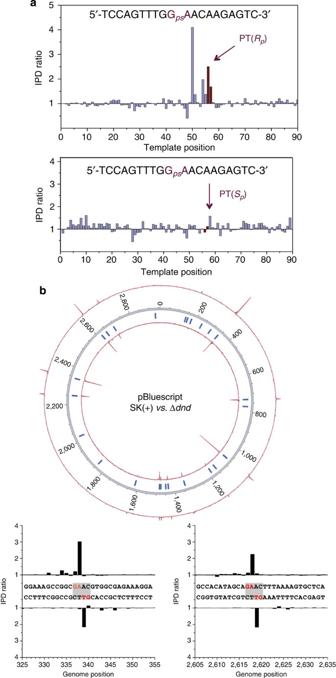Figure 2: Validation of the SMRT method for mapping PT modifications in genomes. To validate the SMRT method, experiments were performed using (a) oligodeoxynucleotides containingSpandRpconfiguration PT modifications and (b) a pBluescript SK(+) plasmid grown inS. entericaserovar Cerro 87 and adndDknockout strain as a control. (a) Upper and lower panels show the kinetic signals for SMRT sequencing of oligodeoxynucleotides containing PT in theRpandSpconfigurations, respectively. (b) Circos plot of kinetic signals of pBluescript plasmids grown inS. entericaserovar Cerro 87 (±PT modification). The inner and outer circles denote IPD ratios for the forward and reverse DNA strands, respectively. Tick marks denote all occurrences of the 5′-GAAC-3′/3′-CTTG-5′ sequence across the plasmid (for IPD ratios at these locations seeSupplementary Table 1). The lower panel shows examples for kinetic signals at two locations on the plasmid. Figure 2: Validation of the SMRT method for mapping PT modifications in genomes. To validate the SMRT method, experiments were performed using ( a ) oligodeoxynucleotides containing S p and R p configuration PT modifications and ( b ) a pBluescript SK(+) plasmid grown in S. enterica serovar Cerro 87 and a dndD knockout strain as a control. ( a ) Upper and lower panels show the kinetic signals for SMRT sequencing of oligodeoxynucleotides containing PT in the R p and S p configurations, respectively. ( b ) Circos plot of kinetic signals of pBluescript plasmids grown in S. enterica serovar Cerro 87 (±PT modification). The inner and outer circles denote IPD ratios for the forward and reverse DNA strands, respectively. Tick marks denote all occurrences of the 5′-GAAC-3′/3′-CTTG-5′ sequence across the plasmid (for IPD ratios at these locations see Supplementary Table 1 ). The lower panel shows examples for kinetic signals at two locations on the plasmid. Full size image At the next level of complexity, the SMRT IPD signature for PT was assessed in plasmid Bluescript SK + extracted from wild-type (WT) S. enterica containing dndB-H and a mutant strain lacking dnd genes. Analysis of the plasmid revealed the expected presence of three common methylated nucleobases: N 6 -methyladenine (m 6 A) in the 5′-G m6 A T C-3′ sequence context, 5-methylcytosine (m 5 C) in 5′-C m5 CW G G-3′ and m 6 A in 5′-CAG m6 AG-3′ (underlined bases indicate methylation on the complementary DNA strand). In addition, extended signatures were detected in the 5′-GAAC-3′/3′-CTTG-5′ sequence context on both DNA strands in the plasmid isolated from WT S. enterica , but not in a PT-free plasmid isolated from the Δdnd -mutant strain, demonstrating that PT modifications were the source of these additional signals ( Fig. 2b , Supplementary Table 1 ). Compared with the PT-induced kinetic signature from oligodeoxynucleotides ( Fig. 2a ), the magnitude of the PT signal in the plasmid was weaker, which was consistent with either sequence-context effects on the SMRT IPD or partial modification of each site in the population of plasmid molecules. To test the latter hypothesis, PT modifications in the plasmid were quantified as PT-linked dinucleotides by liquid chromatography-coupled triple quadrupole mass spectrometry (LC-MS/MS) following nuclease P1 digestion and phosphatase treatment of the plasmid DNA [5] . The presence of 17±0.04 pmol of (G ps T) and 16±0.06 pmol (G ps A) in 18 pmol of plasmid DNA suggested that each plasmid was modified only once on average, implying many 5′-GAAC-3′/3′-CTTG-5′ sites in a given plasmid molecule lacking PT. SMRT sequencing of PT modifications in bacterial genomes Given the ability to detect PT modifications in oligos and plasmid DNA, the SMRT technology was applied to genomic DNA isolated from E. coli B7A and V. cyclitrophicus FF75. As shown in Fig. 3a for B7A, kinetic signatures were detected for the expected m 6 A modifications, as well as signals occurring consistently in the G ps AAC/G ps TTC context. That these new signals were derived from PT modifications is supported (1) by the fact that the observed sequence context is identical to that observed in the plasmid DNA studies from an organism ( S. enterica ) with a nearly identical dnd gene cluster [23] ( Fig. 2b ), (2) by our previous observation of G ps A and G ps T dinucleotide motifs for PT modifications in B7A [5] , and (3) by the identical conclusion reached with the different ICDS approach to PT mapping ( Fig. 1 ), discussed below. 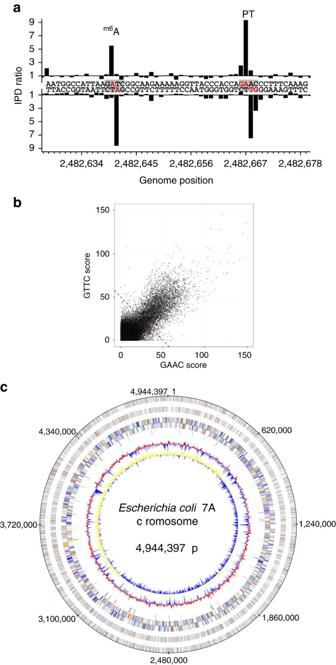Figure 3: Detection of PT by SMRT sequencing across the genome ofE. coliB7A. (a) Example IPD ratio plot showing one instance of PT in a 5′-GAAC-3′/3′-CTTG-5′ sequence context. A nearby adenine methylation signal at 5′-Gm6ATC-3′/3′-CTm6AG-5′ is also shown for comparison. (b) Correlation of opposite DNA strand kinetic signals at 5′-GAAC-3′/3′-CTTG-5′ sites across the B7A genome. The dashed line indicates the threshold for calling sites modified. (c) PT annotation across the B7A chromosome. From outer to inner circles: 1 and 2 (forward, reverse strands): PT sites in ORFs (grey), in non-coding RNA (blue) and non-coding regions (red); 3 and 4: predicted protein-coding sequences coloured according to COG function categories; 5: tRNA/rRNA operons; 6: GC content; 7: GC skew. Figure 3: Detection of PT by SMRT sequencing across the genome of E. coli B7A. ( a ) Example IPD ratio plot showing one instance of PT in a 5′-GAAC-3′/3′-CTTG-5′ sequence context. A nearby adenine methylation signal at 5′-G m6 ATC-3′/3′-CT m6 AG-5′ is also shown for comparison. ( b ) Correlation of opposite DNA strand kinetic signals at 5′-GAAC-3′/3′-CTTG-5′ sites across the B7A genome. The dashed line indicates the threshold for calling sites modified. ( c ) PT annotation across the B7A chromosome. From outer to inner circles: 1 and 2 (forward, reverse strands): PT sites in ORFs (grey), in non-coding RNA (blue) and non-coding regions (red); 3 and 4: predicted protein-coding sequences coloured according to COG function categories; 5: tRNA/rRNA operons; 6: GC content; 7: GC skew. Full size image To analyse the distribution of PT modifications across the B7A genome, we mapped the modifications using the published B7A genome sequence (Genbank ID: AAJT02; annotation in Supplementary Data 1 ) as a reference. Seemingly of importance for an organism in which the PT-modification system ( dndB-E ) is accompanied by a restriction system ( dndF-H ), the PT modifications in B7A were highly biased towards signals on both strands of any given G ps AAC/G ps TTC motif ( Fig. 3b ). Applying a threshold for detection calling from the distribution ( Fig. 3b , dotted line), only ~12% (4855) out of 40,701 GAAC/GTTC sites were detected as modified. The PT modifications were distributed relatively evenly across the B7A chromosome, with an average spacing of ~0.1–10 kb ( Fig. 3c ; Supplementary Data 1 ). We observed a relative underrepresentation of T residues preceding and A and C residues following the G ps AAC/G ps TTC motif, respectively ( Table 1A ). Genome annotation showed that 4499 of 5384 total open reading frames (ORFs), 3 of 86 tRNA genes and 22 of 25 rRNA genes contained at least one PT. The percentage of PT-modified GAAC/GTTC sites in these different regions of the genome varied from 2 to 12%, with 4,499 of 36,607 sites (12%) modified with PT in ORFs, 3 of 118 (2.5%) in tRNAs, 25 of 274 (9.1%) in the rRNAs and 333 of 3702 (9.0%) in the non-coding regions ( Supplementary Data 1 ). Similar frequencies were calculated from the ICDS mapping data ( vide infra , Supplementary Data 2 ), with statistical analyses ( Supplementary Table 2 ) revealing significant under-modification of GAAC/GTTC sites in tRNA genes compared with ORFs and intergenic regions ( P <0.03). This bias against modification in tRNA genes stands in contrast to the observation that the proportion of PT-modified sites varies inversely with the gene length in the B7A genome and that most genes have <4 PT-modified GAAC/GTTC sites ( Supplementary Fig. 1 ). Table 1 Analysis of consensus sequences in E. coli B7A and V. cyclitrophicus FF75* Full size table For the WT FF75 genome, PT was found to occur in the sequence context 5′-C ps CA-3′, while kinetic IPD signatures were absent in the FF75-derived XXL-1 mutant lacking dnd genes ( Fig. 4a,b ; Supplementary Data 3 ). The CCA motif is again consistent with the presence of C ps C dinucleotide observed in FF75 by LC-MS/MS analysis, which occurred at a frequency of 2.6 per 10 3 nt or 6.8-fold higher than the PT modifications in B7A [5] . Interestingly, SMRT sequencing revealed that FF75 possessed PT modifications only on the C ps CA strand, but not on the complementary consensus sequence on the other strand ( Fig. 4 ). This is consistent with the absence of apparent restriction genes in FF75 (by homology searching of the FF75 genome for dndF-H homologs; vide supra ) and with a function for PT modification in FF75 other than a R-M system. Based on the level of SMRT signal noise in the FF75 dnd knockout mutant, we could define the threshold for the IPD kinetic score at a 1% false-positive detection level, translating to 21,778 CCA sites in the WT detected above this threshold, out of a total of 160,541 CCA sites across the FF75 genome ( Supplementary Data 3 ). Mapping the detected modification sites on the genome assembly described above showed that PT-modified CCA was distributed sporadically throughout the genome, with 19,005 located in ORFs, 151 in tRNAs, 761 in rRNA and 1,861 in non-coding regions. There was a preference for A and G following the CCA motif ( Table 1B ). 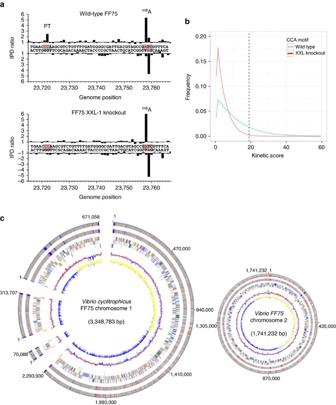Figure 4: Detection of PT by SMRT sequencing acrossV. cyclitrohicusFF75. (a) Example IPD ratio plot showing one instance of PT in a 5′-CCA-3′ sequence context. A nearby adenine methylation signal at 5′-Gm6ATC-3′/3′-CTm6AG-5′ is also shown for comparison. The absence of the PT signal, but not the methylation signal, in the XXL-1 mutant is shown in the lower panel. (b) Kinetic score distributions for the WT and XXL-1 mutant across the FF75 genome. The dashed line indicates the threshold for calling sites modified. (c) PT annotation across the FF75 genome. From outer to inner circles: 1 and 2 (forward, reverse strands): PT sites in ORFs (grey), non-coding RNA (blue) and non-encoding regions (red); 3 and 4: predicted protein-coding sequences colored according to COG function categories; 5: tRNA/rRNA operons; 6: GC content; 7: GC skew. Figure 4: Detection of PT by SMRT sequencing across V. cyclitrohicus FF75. ( a ) Example IPD ratio plot showing one instance of PT in a 5′-CCA-3′ sequence context. A nearby adenine methylation signal at 5′-G m6 ATC-3′/3′-CT m6 AG-5′ is also shown for comparison. The absence of the PT signal, but not the methylation signal, in the XXL-1 mutant is shown in the lower panel. ( b ) Kinetic score distributions for the WT and XXL-1 mutant across the FF75 genome. The dashed line indicates the threshold for calling sites modified. ( c ) PT annotation across the FF75 genome. From outer to inner circles: 1 and 2 (forward, reverse strands): PT sites in ORFs (grey), non-coding RNA (blue) and non-encoding regions (red); 3 and 4: predicted protein-coding sequences colored according to COG function categories; 5: tRNA/rRNA operons; 6: GC content; 7: GC skew. Full size image While the observed signals for m 6 A were consistent in magnitude from previously studied bacteria [27] , the kinetic signals for PT modifications in both B7A and FF75 were more variable, and smaller than what had been determined on the 100% modified oligos ( Figs 2 , 3 , 4 ). The G ps A and G ps T signals in B7A were more pronounced on average than those for C ps C in FF75. There are several potential causes for the lower magnitude in kinetic signals in these bacteria, including partial modification and sequence-context effects on the polymerase IPD kinetic signature. To investigate the former, we analysed the kinetic signals for several genomic positions on a subset of shorter DNA molecules, which allowed the determination of single-molecule PT-modification detection via circular consensus sequencing [32] , [33] . As shown in Fig. 5 for B7A, the analysis shows that underlying the IPD ratio plots averaging over all molecules ( Fig. 5a , left panels) is a heterogeneous composition of DNA molecules that do or do not harbour PT at their respective DNA strand positions ( Fig. 5a , right panels). Conversely, we found genomic locations for which the averaged kinetic signal had not crossed the threshold required for a PT detection assignment, but the single-molecule analysis showed the presence of some DNA molecules harbouring the modification ( Fig. 5b ). This was also observed for FF75 ( Supplementary Fig. 2 ), indicating that the genome-wide PT distribution is partial over these genomes, with varying degrees of PT modifications at the recognition sequence motifs. 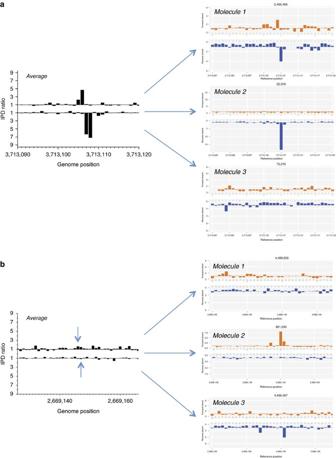Figure 5: Single-molecule analysis suggests partial or incomplete modification of specific sites with PT inE. coliB7A. (a) The kinetic signal average over all molecules at a selected genomic position showing a strong PT kinetic signal is shown on the left forE. coliB7A, with IPD ratio plot examples from single molecules underlying this average, which show between none and full PT-modification signals, are shown on the right. (b) The kinetic signal average over all molecules at a selected genomic position for which there was no detectable PT kinetic signal is shown on the left forE. coliB7A, with IPD ratio plot examples from single molecules underlying this average, which show the presence of some molecules with a PT modification, are shown on the right. Figure 5: Single-molecule analysis suggests partial or incomplete modification of specific sites with PT in E. coli B7A. ( a ) The kinetic signal average over all molecules at a selected genomic position showing a strong PT kinetic signal is shown on the left for E. coli B7A, with IPD ratio plot examples from single molecules underlying this average, which show between none and full PT-modification signals, are shown on the right. ( b ) The kinetic signal average over all molecules at a selected genomic position for which there was no detectable PT kinetic signal is shown on the left for E. coli B7A, with IPD ratio plot examples from single molecules underlying this average, which show the presence of some molecules with a PT modification, are shown on the right. Full size image Development of the iodine-cleavage method for PT mapping As a complement to the SMRT sequencing approach, we developed a method for quantitative localization of PT modifications that exploits the selective reactivity of PT to induce DNA cleavage at the modified phosphodiester linkage [34] . The general concept of the method, which is illustrated in Fig. 1 and in more detail in Supplementary Fig. 3 , involves cleavage of the DNA strand at the site of a PT modification by reaction with iodine in ethanol and subsequent ligation of PCR linkers to the double-strand breaks that result when PT modifications are closely spaced on opposite strands. The iodine-cleavage reaction was validated in two ways. First, matrix-assisted laser desorption ionization time-of-flight mass spectrometry analysis of the cleavage reaction with 48-mer oligodeoxynucleotides revealed that the strand breaks occurred with high efficiency at locations of the PT modification ( Supplementary Fig. 4A ), which is consistent with previous cleavage studies [34] . A second set of control studies entailed treatment of plasmid and genomic DNA possessing and lacking PT modifications, with iodine-cleavage producing strand breaks only in the PT-containing DNA ( Supplementary Fig. 4B,C ). Validation of the method in its entirety was achieved by applying it to genomic DNA isolated from B7A and FF75, as discussed next, with individual DNA manipulation, ligation and amplification steps verified by Fragment Analyzer analysis of DNA fragment sizes. Distribution of PT modifications in E. coli B7A by ICDS Application of the ICDS method to analysis of PT modifications in the B7A genome ( Supplementary Data 2 ) revealed locations that were 90% consistent with the SMRT approach, with mapping data for two independent runs along with a comparison with SMRT data presented in Supplementary Fig. 5 . Sequence motif enrichment analysis was performed on 100 bp regions centred around sites with divergent read pileups using the Motif Elicitation by Expectation Maximisation (MEME)-ChIP algorithmic suite [35] , on sites jointly identified by ICDS and SMRT (4,519 sites), and ICDS only (2,976), respectively. Both data sets displayed a highly significant enrichment for GAAC/GTTC motifs, as expected from the PT enrichment and library construction procedure. The next two motifs (CTGG and G[A/G]TA[A/T]) were also shared by both methods. Analysing the spatial distribution of these motifs revealed that GAAC/GTTC motifs were sharply centred on the middle of the intervals under consideration. While most other motifs did not display any particular localization within the intervals (in spite of being enriched over background), G[A/G]TA[A/T] motifs were significantly underrepresented in the middle of the interval. As evidence of the specificity of ICDS for bistranded PT modifications, application of the method to FF75 produced no detectable PT-modification consensus at CCA, in contrast to the observations with SMRT ( Fig. 4 ) and LC-MS/MS analysis [5] , and despite evidence that iodine cleaves PT in FF75 ( Supplementary Fig. 4C ). Evidence for restriction of plasmid DNA in E. coli B7A We previously demonstrated that a PT-modification-dependent R-M system was present in Salmonella , in which a four-gene cluster ( dptB-E ) was required for PT modification while three additional genes ( dptF-H ) were responsible for restriction [22] . Genome analysis showed that E. coli B7A possessed gene clusters homologous to both the PT modification and restriction gene clusters ( Supplementary Data 1, Fig. 6A,B ). Given the evidence for partial modification of the GAAC/GTTC consensus in E. coli B7A, we analysed the restriction phenotype using WT B7A and a strain lacking the dnd ( dpt -like) gene cluster ( Supplementary Fig. 6A,B ). Equal amounts of pBluscript SK + isolated from E. coli B7A WT (PT-containing DNA) or E. coli B7A ΔdndB-H mutant (DNA lacking PT) were used to test the restriction phenotype of E. coli B7A WT and E. coli B7A ΔdndF-H during transformation. The results of transformation into E. coli B7A WT showed that the plasmid lacking PT had a significantly lower transformation efficiency than PT-containing plasmid ( Supplementary Fig. 6C,D ). However, lack of dndF-H resulted in a similar transformation efficiency for both modified and unmodified plasmids ( Supplementary Fig. 6E,F ). These results suggest that PT modifications in E. coli B7A participate in a restriction-modification system despite the phenomenon of partial modification of the GAAC/GTTC consensus sequence. In vitro PT modification of duplex oligodeoxynucleotides To determine if Dnd proteins could interact directly with a modification consensus sequence, without long-range influences from genomic DNA, we performed an in vitro reaction of a cell-free extract from S. enterica serovar Cerro 87, which has Dnd proteins highly homologous to those in E. coli B7A and a GAAC/GTTC consensus sequence, with a 31-mer duplex oligodeoxynucleotide containing a known GAAC/GTTC-containing PT-modification site from S. enterica [22] ( Supplementary Table 3 ). Following annealing and immobilization of the biotinylated duplex oligo on streptavidin–agarose beads, cell-free extracts were added along with cofactors ATP, L -cysteine and pyridoxal phosphate for a 1-hr reaction, followed by enzymatic release and LC-MS/MS analysis of PT-containing dinucleotides. As shown in Supplementary Fig. 7C,D , assays performed in the absence of oligodeoxynucleotides or cell-free extract did not reveal detectable d(G PS A) or d(G PS T), which rules out contamination from genomic DNA in the cell-free extract. Both d(G PS A) and d(G PS T) were detected in reactions of cell-free extract with a GAAC/GTTC-containing oligodeoxynucleotide ( Supplementary Fig. 7B ), which agrees with the positive control of an oligodeoxynucleotide containing G PS AAC/G PS TTC ( Supplementary Fig. 7A ). These results establish that Dnd proteins directly bind to and react with GAAC/GTTC consensus sequences, which rules out modification systems in which the modification proteins recognize a DNA sequence at a distance from the modification site. Towards the goal of better understanding the biology of PT in bacteria, we surveyed the genomic landscape of PT modifications in two distinct bacteria: E. coli B7A, which possesses an active dndF-H restriction system and V. cyclitrophicus FF75, which lacks dndF-H . Such an analysis required the development of novel convergent technologies to localize PT modifications in DNA, along with complete genomic sequencing for the two bacteria and application of bioinformatic and statistical tools to quantify and localize the PT modifications across the bacterial genomes. To this end, we developed and applied two complementary PT mapping methods: SMRT sequencing technology and ICDS chemical cleavage-based sequencing. As illustrated in Fig. 1 , the SMRT technology involves detection of kinetic signatures when a replicating DNA polymerase encounters modified nucleotides in DNA and has been used to map methylation-based modifications across eukaryotic and prokaryotic genomes [24] , [25] , [26] , [27] , [28] . The oligonucleotide studies revealed a fortuitous bias by the polymerase towards PT modifications in the naturally occurring R p configuration on the template, while the plasmid studies not only demonstrated detectability of the GAAC/GTTC motif that would be observed in B7A but also suggested a phenomenon of partial modification of any specific GAAC/GTTC site in the plasmid. While neither the SMRT nor the ICDS method can rule out PT modification at a site, two facts prove that the Dnd proteins do not incorporate PT at every available site in every plasmid: (1) LC-MS/MS analysis revealed that PT modifications occurred once per plasmid molecule on average; and (2) PT signals were only clearly detected at ~15 of 25 GAAC/GTTC sites ( Supplementary Table 1 ) in a population of plasmid molecules. Hence, the definition of a partial modification phenomenon, which appears to be the case in bacterial genomes as discussed shortly. As a complement to SMRT sequencing, the ICDS method is based upon creating a double-strand break at sites containing PT modifications in close proximity on opposite DNA strands, and is thus limited to genomic mapping of bistranded PT modifications as in B7A but not the single-stranded modifications in FF75. The iodine-based chemical cleavage of PT-containing DNA nonetheless serves as a rapid assay for the presence of PT modifications, analogous to the cleavage phenomenon that occurs during agarose gel electrophoresis [23] . The feasibility of the ICDS method was demonstrated in not only oligodeoxynucleotides but also plasmid and genomic DNA ( Supplementary Fig. 4 ), and its specificity for bistranded PT modifications evident in the lack of detectable signal with FF75 DNA compared with the clear GAAC/GTTC consensus observed in B7A. Unlike the consistency and magnitude of the IPD ratio for m 6 A (ref. 27 ), the kinetic signals for PT modifications in both B7A and FF75 were variable and smaller than m 6 A signals ( Figs 3 , 4 ), with the G ps A and G ps T signals in B7A larger on average than those for C ps C in FF75. There are several explanations for this variation in IPD kinetic signals. First, it is possible that the flanking regions of a PT-modification site could affect the polymerase and alter the IPD, with some IPD signals falling below the detection limit of the system. Alternatively, PT modification does not occur consistently at a given site in a genome in a population of bacteria—the phenomenon of partial modification. It is also possible that hemimodification of the GAAC/GTTC motif occurs, as suggested by the lack of PT signal on one strand of some modification sites in B7A ( Fig. 5 ; Supplementary Data 1 ), although this appears to be a low-frequency phenomenon given the quantitative concordance of the SMRT and ICDS data ( Supplementary Fig. 5 ). In the case of partial modification, the aggregate kinetic data would represent ensembles of signatures for both modified and unmodified cases. The fact that LC-MS/MS analysis revealed fewer PT modifications than modification sites in the plasmid studies ( Fig. 2 ) suggests that partial modification is operant in B7A, which poses a problem given the presence of a restriction system in B7A ( Supplementary Fig. 6 , see below). The PT mapping methods were next applied to the genomes of B7A and FF75. PT modification in B7A was determined by both SMRT and ICDS to occur in the G ps AAC and G ps TTC sequence context, which is consistent with the previous observation of equimolar quantities of d(G ps A) and d(G ps T) detected in the genome by LC-MS/MS [5] . Both the complementarity of the d(G ps A) and d(G ps T) dinucleotides in the context of a GAAC/GTTC motif and the clear observation of PT modifications on both strands at a GAAC/GTTC sequence prove that PT occurs predominantly as a bistranded DNA modification in B7A ( Fig. 3 ). Although the frequency of PT modifications in GAAC/GTTC motifs (~1 per 3,000 nt) suggested a ~6 nt consensus sequence [5] , as might be expected for a classical type II R-M system, analysis of the flanking sequences out to 100 nt on either side of all PT-modification sites revealed by both SMRT and ICDS revealed no apparent strict consensus beyond GAAC/GTTC. Indeed, only 12% of 40,701 possible GAAC/GTTC sites were modified in B7A, which is similar to the observation of 14% PT modification of 160,541 possible CCA sites in FF75, yet there are no clear sequence determinants for PT modification at these sites. The results raise questions about how Dnd modification proteins (DndA-E) select their DNA targets. While it is not known which Dnd protein selects the DNA binding site, emerging evidence suggests that DndD is a DNA nicking enzyme and that DndE binds selectively to nicked DNA, with both activities critical to incorporation of PT into the DNA backbone. [19] That the Dnd proteins directly bind to and modify a GAAC/GTTC-containing sequence is established in our in vitro oligodeoxynucleotides PT-modification studies using cell-free extracts ( Supplementary Fig. 7 ) and suggests that one or more of the Dnd proteins possess a GAAC/GTTC recognition element. However, it is still unclear why only 18% of all GAAC/GTTC sites are modified, except to say that there must be other features of local DNA structure that are not amenable to a discrete consensus sequence but are targeted by Dnd proteins. Alternatively, the physiology of the dnd -based R-M system may balance less-than-saturating modification densities across the genome with a restriction system that does not depend upon saturation with PT modifications, as discussed shortly. Another mechanism for exclusion of some GAAC/GTTC targets for modification in B7A involves the observation that PT modifications rarely occur at TGAACA motifs (35 out of 3785 sites; Table 1 ). It is possible that this particular sequence has a function that obviates modification by PT in B7A. One such function may involve binding of regulatory proteins. The strongest evidence for this model arises from the binding sites for torR [30] and rpoE (sigmaE factor) [36] . TorR is the response regulator (OmpR/PhoB family) of the tor CAD operon that encodes the trimethylamine N-oxide alternative respiratory system and its DNA binding consensus (CTGTTCATAT) contains the low-modified TGTTCA motif [30] ( Table 1 ). Similarly, RpoE/sigmaE factor controls transcription of stress response genes such as heat shock proteins and has a binding consensus of GAACTT followed by A and TCTRA 12 and 18 nt downstream [36] . The presence of these rare GAAC/GTTC motifs in the binding sites of important regulatory proteins is consistent with a model in which the PT-modification system avoids incorporating PT at the binding consensus site. It is also possible that the presence of the regulatory protein bound at the non-modified consensus could protect the unmodified site from cleavage by the PT-dependent restriction system. Furthermore, an analysis at the online database, REBASE, for restriction recognition sequences that include GAAC/GTTC revealed eighteen total, but only two known enzymes, UbaPI (CGAACG) and DrdII (GAACCA), overlap significantly with PT-modification sites identified in B7A, and yet both lack known cleavage sites, still allowing for a possible concurrence of recognition. This suggests that the PT-modification system does not compete or interfere with other known restriction-modification systems. Another intriguing feature of PT-modification biology that arises from our studies is the apparent conundrum of partial modification of specific GAAC/GTTC sites in the presence of a PT restriction system. The presence of dndF-H in B7A and our evidence for restriction activity ( Supplementary Fig. 6 ) prove that PT modifications in B7A are part of an R-M system. However, it is clearly not a type II R-M system with a clearly defined consensus sequence. Further, the evidence from SMRT single-molecule analysis for less than full penetration of PT modification at a specific genomic site in all bacteria in a population suggests that the simple lack of a PT modification at a potential modification site does not make the sequence susceptible to cleavage by the restriction protein(s). This partial modification phenomenon is consistent with our previous observation that over-expression of DndA-E proteins increases the level of PT modifications in a dose-dependent fashion, with retention of the same dinucleotide sequence contexts. [5] This is consistent with either an increase in the efficiency of modification of any particular site or the modification of new sites containing the core consensus sequence. These results point to a novel R-M system involving site-specific PT modifications without a predictable consensus beyond four nucleotides and with partial modification of sites in the presence of a restriction activity. One of many possible explanations for this partial modification phenomenon involves a similar behaviour in certain type III methyltransferase systems, in which cell populations can be a mixture between states in which the methyltransferase is active or inactive. In some cases, ~1% of the cells have the methyltransferase turned on (that is, SMRT sequencing would detect the methylation) while 99% of the cells have the methyltransferase turned off [37] . A similar phenomenon could explain the appearance of sites only partially modified with PT in the bacterial population when the ensemble is analysed by SMRT and ICDS sequencing. The mapping of PT modifications across the FF75 genome also revealed novel features of PT biology. In sharp contrast to B7A, PT modification in FF75 occurred as a single-stranded modification ( Fig. 4 ) at CCA motifs, which is again consistent with LC-MS/MS evidence of only a d(C ps C) dinucleotide motif in FF75 (ref. 5) [5] . The previous quantitation of d(C ps C) at 1 modification per ~380 bp suggested a 4 nt consensus sequence. Alignment of 40 nt of surrounding sequences revealed no strict further sequence-context constraint beyond the 3-nt C ps CA context, although the fourth base showed a strong bias against T, and a moderate preference towards A or G ( Table 1B ). In addition, no dndFGH homologue was found in FF75. Single-molecule analysis revealed that CCA sequences in genomes are also dynamically PT modified ( Supplementary Fig. 2 ). Based on the features of single-strand modification and absence of dndFGH restriction genes, we conclude that the PT modifications in FF75 play a biological role other than R-M. Using two novel genome-sequencing methods, PT modifications were mapped across the genomes of two bacteria, which revealed the identification of bistranded PT modifications at GAAC/GCCT sites in B7A and single-strand modifications at CCA in FF75, with no wider consensus sequence apparent, only 12–14% of all GAAC/GCCT sites modified, and less than full modification of any particular site across all bacteria in a population. Such consistency for two bacteria in which PT has very different functions points to a conserved mechanism of DNA target selection by the DNA-modifying DndA-E proteins, a mechanism that we have shown likely involves direct interaction of the modifying proteins with the consensus sequence. PT modifications in B7A are clearly not part of a type II R-M system, but also lack the predictive modification consensus sequences and the completely saturated modification sites associated with type I, III and IV R-M systems. Furthermore, the results with FF75 point to PT functions other than R-M. For example, one alternative function might involve epigenetic control of gene expression, as illustrated by non-R-M methylation-based DNA modifications in many bacteria. Materials and bacterial strains Enantiomerically pure d(G ps A) and d(G ps T) in R p and S p configuration were obtained from IBA Bio-Tagnology (Germany). Oligodeoxynucleotides containing PTs were synthesized by Sangon Biotech Co. Ltd. (Shanghai). The plasmid pBluescript SK(+) was obtained from Life Technologies (Grand Island, NY). Salmonella enterica serovar Cerro 87 was supplied by Professor Toshiyuki Murase (Tottori University, Japan), E. coli strain B7A was obtained from Dr Jaquelyn Fleckenstein (Departments of Medicine and Molecular Sciences, University of Tennessee Health Science Center) [4] , [5] , Vibrio cyclitrophicus FF75 was obtained from Prof. Martin Polz (Massachusetts Institute of Technology, Cambridge, MA, USA) [5] . The following kits were purchased from Qiagen (Hilden, Germany): QIAGEN Genomic-tip 500/G, DNA Maxi Kit (Blood & Cell Culture) and QIAquick PCR Purification Kit. The following kits and reagents were purchased from New England BioLabs (Ipswich, MA): Antarctic Phosphatase, Quick Blunting Kit, Quick Ligation Kit, Klenow Fragment (3′→5′ exo − ), dATP solution and HindIII. Custom oligodeoxynucleotides were ordered from Integrated DNA Technologies (Coralville, IA) and Sangon Biotech Co. Ltd. (Shanghai) (sequences shown in Supplementary Table 3 ). Centrifugal filters (10k MWCO) were from VWR International (Radnor, PA) and MicroSpin G-25 columns were from GE Healthcare (Buckinghamshire, UK). Iodine and 3-hydroxypicolinic acid (MALDI matrix) were from Sigma-Aldrich (St Louis, MO). PCR tubes were from Molecular BioProducts (San Diego, CA). All water was deionized and filtered using a MilliQ water purification system (EMD Millipore, Billerica, MA). Isolation of plasmids and genomic DNA The plasmid pBluescript SK(+) for SMRT sequencing was extracted from WT S. enterica serovar Cerro 87 and from its mutant lacking the dnd gene cluster [22] , both grown in Luria-Bertani (LB) medium in 16 h cultures using the Genomic-tip 500/G kit. Overnight cultures of E. coli B7A in LB were diluted and regrown to an O.D. (600 nm) of ~2 to achieve a logarithmic phase of growth. Genomic DNA was isolated using three 500/G columns as outlined in the Qiagen DNA Maxi Kit. Vibrio strains were grown at 28 °C in tryptic soy broth medium supplemented with 2% NaCl and DNA isolated by standard protocols. Preparation of E. coli B7A ΔdndFGH The mutant B7A ΔdndFGH was constructed by homologous recombination using thermo- and sucrose-sensitive plasmid pKOV-Kan. Total DNA from E. coli B7A was used as a template to amplify the left and right arms of the dnd cluster ( dndB-H ), introducing BamHI and SalI restriction sites flanking dndF-H . Primers for the 611-bp left arm were B7A-FLL (sequence in Supplementary Table 3 ) and B7A-FLR; for the 643-bp right arm were B7A-HRL and B7A-HRR (SalI site underlined in Supplementary Table 3 ). The left and right arms were amplified together, overlapping by 40 bp. Primers B7A-FLL and B7A-HRR were used for the 1254-bp recombinant fragment with introduced BamHI and SalI sites. The entire homologous recombination region was cloned into the plasmid pKOV-Kan, cleaved with BamHI and SalI to release dndFGH and religated to generate pJTU6601. The pJTU6601 was introduced by transformation into E. coli DH10b harbouring a plasmid containing dndB-E (pJTU1238) to allow phosphorothioation of the pJTU6601 plasmid DNA. The PT’d pJTU6601 was then introduced into E. coli B7A at 30 °C. The single crossover intermediate (ZXQ-1) was obtained at 43 °C and the double crossover (B7A ΔdndFGH ) was obtained on a plate containing 15% sucrose at 43 °C. Primers B7A-FLL-L and B7A-HRR-R were used for screening the single crossover, and B7A-T1 and B7A-T2 (primer sequences in Supplementary Table 3 ) were used for screening the double crossover ( Supplementary Fig. 3 ). Characterization of the restriction activity in E. coli B7A PT-modified and PT-free plasmids (pBluescript SK(+)) were isolated from WT E. coli B7A and its Δ dndB-H mutant strain, respectively, and were purified using the GenElute plasmid miniprep kit (Sigma) and quantified by absorbance at 260 nm. Electrocompetent E. coli B7A cells were prepared using a standard protocol with a 10% glycerol wash and electroporation was performed with a Micropulser (Bio-Rad) according to manufacturer’s instructions using 10 ng of plasmid DNA and 40 μl of cells. Electroporated cells were incubated in 1 ml of SOC medium at 37 °C for 1 h and then plated onto LB agar medium containing antibiotic to select for transformed colonies. Preparation of PT-containing oligonucleotides An oligonucleotide ( Supplementary Table 3 ; PT-S4) containing a PT-modified G ps AAC motif was chemically synthesized and R p and S p PT configurations of this oligo were fractionated by reversed-phased HPLC on an Agilent 1210 series system with an Agilent TC-C18 column (4.6 × 250 mm, 5 μm particle size) at a flow rate of 1 ml min −1 with the following parameters: column temperature: 45 °C; solvent A: 0.1 M NH 4 OAc; solvent B: 20mM NH 4 OAc in 80% acetonitrile; gradient: 3% B for 10 min, 3% B to 15% B over 40 min; 95% B for 10 min; detection by UV absorbance at 260 nm. Quantification of PT modifications in DNA PT modifications in plasmid pBluescript SK(+) isolated from E. coli B7A were quantified by liquid chromatography-coupled, time-of-flight mass spectrometry as the dinucleotides d(G ps A) and d(G ps T), essentially as described elsewhere [5] . Plasmid DNA was hydrolyzed with nuclease P1 (Sigma; 2 U) in 30 mM sodium acetate, pH 5.3, 0.5 mM ZnCl 2 in a 100 μl volume at 50 °C for 2 h. Subsequent dephosphorylation was carried out by the addition of 10 μl of 1 M Tris-Cl, pH 8.0 and 5 U of alkaline phosphatase (Fermentas, FASTAP) at 37 °C for another 2 h. The enzymes were subsequently removed by ultrafiltration (AMICON ULTRA 0.5 ml Ultracel 3 kD) followed by the addition of 100 pmol of d(G ps A) S p as an internal standard. The digested DNA sample was dried and resuspended in 20 μl of deionized water for quantification by liquid chromatography-coupled, time-of-flight mass spectrometry analysis against external calibration curves for d(G ps A) S p , d(G ps T) R p , and d(G PS A) R p . The digestion mixture containing PT dinucleotides was resolved on an Agilent SB-C18 column (150 × 2.1 mm, 3.5 μm particle size) with a flow rate of 0.3 ml min −1 and the following parameters: column temperature: 35 °C; solvent A: 0.1% acetic acid; solvent B: 0.1% acetic acid in acetonitrile; gradient: 3% B for 5 min, 3% to 15% B over 20 min, and 15% to 100% B over 1 min. The HPLC column was coupled to an Agilent 6410 QTOF mass spectrometer with an electrospray ionization source in positive mode with the following parameters: gas flow, 10 l min −1 ; nebulizer pressure, 30 psi; drying gas temperature, 325 °C; and capillary voltage, 3,100 V. Multiple reaction monitoring mode was used for detection of product ions derived from the precursor ions, with all instrument parameters optimized for maximal sensitivity (retention time in min, precursor ion m/z, product ion m/z , fragmentor voltage, collision energy): d(G ps A), 20.5, 597, 136, 120 V, 40 V; d(G ps T), 26.5, 588, 152, 110 V, 17 V. Library preparation and SMRT sequencing SMRTbell sequencing templates were prepared as described previously [38] . B7A and FF75 gDNA was fragmented to either 500–800 bp using adaptive focused acoustics (Covaris; Woburn, MA, USA) or an average size of ~10 kb using gTUBES (Covaris). Fragmented DNA was end-repaired, ligated to hairpin adaptors and incompletely formed SMRTbell templates were digested with a combination of Exonuclease III (New England Biolabs; Ipswich, MA, USA) and Exonuclease VII (Affymetrix; Cleveland, OH, USA). SMRT sequencing was carried out on the PacBio RS (Pacific Biosciences, Menlo Park, CA, USA) using C2 chemistry with 2 × 45 min movies for the small insert libraries or XL/C2 chemistry with one 90 min movie for the large insert libraries. Genome assembly B7A and FF75 genomes were assembled using HGAP [30] with default parameters in the SMRT Analysis Suite version 1.3 (Pacific Biosciences, Menlo Park, CA, USA). Additional manual assembly of contigs was carried out in cases of unique overlapping sequence. Consensus sequence polishing was done with Quiver version 1.3. Detection of PT modifications in SMRT sequencing data Base modification analysis was performed using the base modification detection workflow of SMRT Analysis version 1.3. The single-molecule base modification analysis used to query the underlying heterogeneity of modifications across individual molecules is analogous to the standard base modification analysis supported in SMRT Analysis. In the standard method, the IPD ratio per given position is calculated by averaging the IPD values across all the subreads from multiple molecules before comparing with the in silico control IPD. In the single-molecule method, only the subreads from an individual molecule are used for the IPD ratio calculations for the given molecule (reads were filtered for having five or more subreads, and required three or more IPDs with the preceding and following base correct for computation of the single-molecule IPD ratio). Iodine-cleavage deep sequencing of PT modifications As illustrated in Fig. 1 and Supplementary Fig. 3 , closely opposed, bistranded PT modifications were mapped in DNA by exploiting iodine-induced DNA strand cleavage at sites containing by PT [34] , [39] , [40] and then performing double-stranded ligation of a sequencing linker followed by Illumina sequencing. The first step of the ICDS method involves iodine cleavage at genomic PT sites. Immediately before iodine treatment, 21 μg of gDNA was diluted to 500 μl with water and re-concentrated (repeated 5 × ) using a 10k MWCO centrifugal filter to remove any contaminating Tris buffer. A 30 mM iodine solution in ethanol was freshly prepared and reactions (60 μl) were then setup in PCR tubes as follows: gDNA (10.5 μg), 50 mM Na 2 HPO 4 , pH 9.0, 3 mM I 2 or 10% ethanol (carrier control) [39] , [40] . Using a thermal cycler (MJ Research PTC-200), reactions were heated to 65 °C for 5 min and then slow cooled (0.1 °C s −1 ) to 4 °C and then placed on ice. Residual iodine (or ethanol) and salts were then removed using MicroSpin G-25 columns. To confirm the specificity of iodine cleavage, three separate experiments were performed using site-specific PT modifications in oligodeoxynucleotides, PT in plasmids and PT in gDNA. First, complementary 48-mer oligodeoxynucleotides, each containing a single PT modification ( Supplementary Table 3 ), were subjected to an iodine-cleavage reaction and products were characterized by matrix-assisted laser desorption ionization time-of-flight mass spectrometry ( Supplementary Fig. 4A ). In a second study, plasmids with (pBluescript SK(+) harvested from WT E. coli B7A) and without (pBluescript SK(+) from E. coli B7A Δ dndB-H ) PT modifications [5] were subjected to iodine cleavage and a portion of each sample was subsequently treated with HindIII to linearize the plasmids, and samples run on a 1% agarose gel with 1 × TBE ( Supplementary Fig. 4B ). Finally, in a third experiment, gDNA from FF75 with (wild type) and without (XXL-1) PT modifications and gDNA from B7A with (wild type) and without (Δ dndB-H ) PT modifications were subjected to iodine cleavage and samples were run on a 0.7% agarose gel with 1 × TBE ( Supplementary Fig. 4C ). Following iodine cleavage, the DNA was subjected to end-processing and tag ligation at double-strand break sites. Cleaved gDNA samples (including an ethanol control) were processed as follows, according to instructions provided with the NEBNext DNA Library Prep Reagent Set for Illumina (New England BioLabs, Beverly, MA). Terminal phosphates were removed with Antarctic Phosphatase (10 units) at 37 °C for 60 min. To inactivate the enzyme, a thermal cycler (MJ Research PTC-200) heated the samples to 65 °C for 10 min and then slow cooled them (0.1 °C s −1 ) to 4 °C to assure proper complementary re-annealing. Break sites were blunt-ended using the Quick Blunting Kit at 22 °C for 30 min. The thermal cycler-heated samples to 75 °C for 12 min to inactivate the enzymes and then slow cooled as before. Samples were cleaned up using QIAquick columns and eluted with 32 μl elution buffer and 10 μl water. Next, blunt-ends were 3′-deoxyadenylated (that is, A-tailing) in reactions (63 μl) containing 1x NEBuffer #2, 20 mM dATP, and Klenow (3′→5′exo − ) (15 units) at 37 °C for 30 min. The thermal cycler-heated samples to 70 °C for 20 min and then slow cooled. Samples were cleaned up using QIAquick columns and eluted with 32 μl elution buffer and 10 μl water. Finally, a custom 20-mer duplex tag-sequence ( Supplementary Table 3 ; 5′-FWD tag/3′-REV tag) (3 μM) was ligated to 3′-deoxyadenylated ends using the Quick Ligation Kit at 22 °C for 10 min. The thermal cycler-heated samples to 75 °C for 12 min and then slow cooled. Samples were cleaned up using QIAquick columns and eluted with 100 μl water. The gDNA was then sonicated with a Branson Sonifier (S-250A) equipped with a Big Horn amplifier and a 1/8” tapered micro-tip probe to fragment the gDNA to achieve an optimal range (150–350 bp) for subsequent Illumina sequencing. Samples were diluted to 800 μl with water and subjected to energy pulses (50% duty cycle) for 12 min total (2 min ON, 1 min OFF) × 6, while on ice to avoid excessive heat. An output setting of 1.3 yielded a reading of ~20 on the metre. After sonication, samples were concentrated on a SpeedVac system to ~50 μl and submitted for further processing and Illumina sequencing. The fragmented DNA was finally subjected to Illumina sequencing, with 1.1 ng of iodine fragmented gDNA and 38.3 ng of mock (EtOH) fragmented DNA ligated to standard Illumina paired-end adaptors using the SPRIworks Fragment Library System (Beckman Coulter Genomics) and size selected for inserts between 150 and 350 nt. Ligated products were amplified 15 cycles (iodine treated) and 19 cycles (control) using Paired-End PCR Primer 1.0 and 15-TACCGC PCR Primer 2.0 or 16-ATGATA PCR Primer 2.0, respectively ( Supplementary Table 3 ), in order to introduce custom second read sequencing primers and molecular barcodes (TACCGC for iodine-treated and ATGATA for ethanol control). Completed libraries were quantified using qPCR compared with known standards and Fragment Analyzer analysis (Advanced Analytical). Quantified libraries were multiplexed and loaded on an Illumina GAIIx sequencer at 5 pM. The Illumina libraries were run alongside a PhiX control lane on a two-lane partial flowcell run (42) with 25 nt read on the first read, 6 nt read in the barcode and 45 nt read on the reverse read after paired-end turnaround and priming with the Custom Paired-End Read 2 reverse primer on the sample lane. Cluster identification and base calling was performed using the Illumina RTA package (1.13.48) using the PhiX lane as a control for base intensity. Sequencing reads were mapped against the Pacific Bioscience-based E. coli B7A genome assembly using Bowtie2.0 version 2.1.0 in paired-end mode (options—p 2–D 15–R 2–N 0–L 22–i S,1,1.15) [41] . Mapping statistics are summarized in Supplementary Table 4 . Sorted bam files were generated with samtools v 0.1.16 (r963:234) and indexed [42] . Alignments were visualized using the Integrative Genome Viewer, version 2.3.8 (ref. 43) [43] . To assess genome coverage and read pileup overlaps, sequencing depths were computed for each sample at each position across the B7A genome using bedtools (v2.16.1) coverage—d for each strand separately [44] . Resulting coverage maps were postprocessed to extract regions with coverage deeper than set thresholds (typically 100, 150 and 200 reads per position), and overlaps of such regions were identified using bedtools intersect. Divergent read pileups were identified by extending the region 50 bp upstream of the 5′ most boundary of the read pileup on the corresponding strand. The detailed strategy to fine-map PT modifications is summarized in Supplementary Fig. 5 . All individual read start positions were recorded for both strands, and starting positions shared by 50 or more reads were retained for analysis. Regions where starting positions mapped within 8 bp on opposite strands were verified not to be enriched in the control sample (as defined by no positions with 50 or more reads starting within the 8 bp window in the ethanol-treated control sample). Finally, read starting sites mapping within less than 3 bps were collapsed into the centremost 8 bp region, which were used for the final call of PT sites. Overlaps with SMRT-defined sites and known locations of GAAC/GTTC sites in the B7A genome were also computed with bedtools. Genomic regions falling under read pileups of interest were queried using bedtools bedToFasta. An online implementation of the MEME tailored to large-scale genomic data (MEME-ChIP 4.9.0, http://meme.nbcr.net/meme/cgi-bin/meme-chip.cgi ; [35] ) were used for motif identification under read pileups, using parameters –time 120 –db db/dpinteract.meme -meme-mod anr -meme-minw 4 -meme-maxw 30 –meme-nmotifs 10 –dreme-e 0.05 –centrimo-score 5 –centrimo-ethresh 10. Motifs were queried using the DREME component of the suite [45] , and their spatial localization was assessed using CENTRIMO, allowing for the identification of motifs peaking away from the centre of the interval. In addition, the same sequences were subjected to motif enrichment analysis based on a first-order Markov Model (1MM), adapted fromref. [46] . Sequences were divided into equally sized bins according to their G and C nucleotide composition (%GC). Using the same sequences, background mono- and di-nucleotide frequencies were computed to build a first-order Markov model (1 MM) of the sequences in each bin. Background probability of a hexamer was calculated per bin and averaged to get the overall background probability. The actual frequency of a hexamer was obtained by counting its occurrences in all sequences extracted from read pileups. Statistical analysis of SMRT and ICDS PT mapping data Candidate PT-modified sites called from both methods were mapped with respect to genomic annotations reported in Supplementary Data 1 using bedtools. Pairwise comparisons between the number of sites mapping to genomic features were performed using a λ 2 test for each method/run individually, and P -values were adjusted for multiple testing using the Benjamin–Hochberg procedure. A Haenzsel–Mantel test was performed to interrogate biases in number of PT-modified sites between genomic features across all three methods/runs, and pooled odds ratios were calculated using the mantelhaen.test in the R 2.11.1 stats package. In addition, Student's t -tests were used to compare average numbers of PT-modified sites between genomic features across all methods/runs. Reaction of oligonucleotides with cell-free extract and analysis of PT A cell-free extract was prepared from S. enterica serovar Cerro 87 by growing cells in 200 ml of LB medium at 37 °C to an A 600 of 1.5, followed by harvesting the bacteria (centrifugation 5,000 g , 10 min, 4 °C), washing the cells three times with phosphate-buffered saline (PBS) (4 °C), and resuspending the pellet in 20 ml of lysis buffer (20 mM Tris-HCl, pH 8.0, 60 mM KCl, 10 mM MgCl 2 , 1 mM EDTA, 2 mM DTT, 1 mM PMSF and 25% glycol). Resuspended bacteria were subjected to three complete cycles of freeze–thawing and disruption by sonication, with the soluble protein from the cell lysate collected in the supernatant after centrifugation (15,000 g , 20 min, 4 °C). Duplex biotinylated oligodeoxynucleotides substrates ( Supplementary Table 3 ) were prepared by annealing complementary strands (100 pmol μl −1 in 200 μl of water) at 95 °C for 5 min followed by cooling to ambient temperature. The duplex oligodeoxynucleotides (10 μl of 10 pmol μl −1 ) were then incubated with 100 μl of streptavidin–agarose beads (Sigma Chemical; washed three times with 1 ml PBS) for 2 h at 25 °C to allow the biotin–streptavidin reaction to occur, followed by washing the bound beads three times with PBS (centrifugation 800 g , 4 °C, 1 min). The bead-bound oligodeoxynucleotides were then used in phosphorothioation reactions with cell-free extract. The standard reaction consisted of 100 pmol equivalents of biotinylated oligonucleotides bound to agarose beads, 2.5 mM ATP, 1 mM L -cystiene, 0.1 mM pyridoxal phosphate and 1 ml cell extract and was incubated at 25 °C for 2–3 h. The bead-bound oligodeoxynucleotides were then washed three times in 1 ml of PBS (centrifugation 800 g , 1 min, 25 °C) and the oligodeoxynucleotides (100 pmol in 100 μl) digested 4 U of nuclease P1 in 30 mM sodium acetate, pH 5.2, 0.5 mM ZnCl 2 in 200 μl total volume at 37 °C for 2 h. The resulting 2-deoxynucleotides and PT-linked dinucleotides were dephosphorylated by the addition of 17 U of alkaline phosphatase and 20 μL of 1 M Tris-Cl, pH 8.0 and incubation at 37 °C for 2 h. The enzymes were subsequently removed by ultrafiltration (YM-10 column; Microcon). d(G PS A) and d(G PS T) dinucleotides were then quantified by HPLC-coupled tandem mass spectrometry (LC-MS/MS). Chromatographic separation was achieved using a Agilient ZORBAX SB-C18 column (150 × 2.1 mm, 3.5 μm particle size) with elution at 35 °C and a flow rate of 0.3 ml min −1 using a gradient of 97% buffer A (0.1% acetic acid in water) and 3% buffer B (0.1% acetic acid in acetonitrile) for 5 min, followed by 3% to 15% buffer B over 20 min and 15 to 100% buffer B over 1 min. The HPLC column was coupled to an Agilent 6410 mass spectrometer with an electrospray ionization source in positive mode with the following parameters: gas flow, 10 l min −1 ; nebulizer pressure, 30 psi; drying gas temperature, 325 °C; and capillary voltage, 3,100 V. Multiple reaction monitoring modes were used for detection of product ions derived from the precursor ions, with all instrument parameters optimized for maximal sensitivity (retention time in min, precursor ion m/z , product ion m/z , fragmentor voltage, collision energy): d(G PS A), 20.5, 597, 136, 120 V, 40 V; d(G PS T), 26.5, 588, 152, 110 V, 17 V. How to cite this article : Cao, B. et al . Genomic mapping of phosphorothioates reveals partial modification of short consensus sequences. Nat. Commun. 5:3951 doi: 10.1038/ncomms4951 (2014). Accession codes : The contigs, annotated by RAST, for Vibrio cyclitrophicus FF75 have been deposited in the GenBank/EMBL/DDBJ nucleotide core database under the accession code ATLT00000000 .